Short-lived charge-transfer excitons in organic photovoltaic cells studied by high-field magneto-photocurrent The main route of charge photogeneration in efficient organic photovoltaic cells based on bulk hetero-junction donor–acceptor blends involves short-lived charge-transfer excitons at the donor–acceptor interfaces. The cell efficiency is critically affected by the charge-transfer exciton recombination and dissociation processes. By measuring the magneto-photocurrent under ambient conditions at room temperature, we show here that magnetic field-induced spin-mixing among the charge-transfer exciton spin sublevels occurs in fields up to at least 8.5 Tesla. The resulting magneto-photocurrent increases at high fields showing non-saturating behaviour up to the highest applied field. We attribute the observed high-field spin-mixing mechanism to the difference in the donor–acceptor g -factors. The non-saturating magneto-photocurrent response at high field indicates that there exist charge-transfer excitons with lifetime in the sub-nanosecond time domain. The non-Lorentzian high-field magneto-photocurrent response indicates a dispersive decay mechanism that originates due to a broad distribution of charge-transfer exciton lifetimes. The spin degree of freedom plays an important role in the photo-physical processes of organic photovoltaic (OPV) cells based on donor–acceptor (D–A) hetero-junction blends, which contain separate donor and acceptor intertwined nano-sized domains [1] . For example, weakly bound polaron pairs (PP) at the D–A interfaces allow singlet/triplet spin-mixing that affects charge recombination loss, which consequently suppresses the device efficiency. In addition, it is now clear that the main route of the charge photogeneration process that starts from photo-excited singlet excitons (SEs) in the polymer donors involves an intermediate state of charge-transfer exciton (CTE) at the D–A interfaces that either recombines or dissociates into free polarons in sub-nanosecond time [2] . The CTE comprises a tightly bound PP across the interface of negatively charged polaron (P − ) on the acceptor and positively charged polaron (P + ) on the donor. The CTE and SE species can be distinguished by their characteristic exchange coupling, J . For SE in π-conjugated polymers, J may be as large as 0.4 eV, whereas J is exceedingly small for CTE and PP due to their ionic nature having negative and positive charges on different molecules. The efficiency of OPV cells critically depends on the ability of the photogenerated SE in the donor polymer domain to reach the D–A interface forming CTE, before fast recombination sets in. Moreover, on a longer timescale the cell photocurrent (PC) is also determined by the ability of the CTE to ionize (dissociate) into positive and negative free charge carriers (polarons). Alas, polaron recombination also happens on a much longer timescale through loosely bound PP at the D–A interfaces. Since the D–A blend is in general of amorphous structure, the P + --P − size is not constant across the various interfaces, and this may provoke a distribution of binding energies and recombination rates. There exist a number of spin-dependent recombination processes in organic semiconductors that are influenced by various spin-mixing processes controlled by external factors, such as material composition, morphology and magnetic field. We emphasize in this work several relevant spin-mixing mechanisms, which are: (a) spin-mixing by the hyperfine interaction (HFI) within the PP species [3] , [4] , [5] , [6] , [7] ; and (b) spin-mixing in PP and CTE via the difference, Δ g , in the electron and hole g -factors in blends of organic semiconductors and fullerene [8] , [9] . In addition to these ‘non-equilibrium’ spin-mixing mechanisms, we also discuss the effect of spin polarization in high magnetic fields under thermal equilibrium conditions [10] , where the spin lattice relaxation rate is much larger than the PP recombination rate. The amorphous nature of the D–A blend in bulk hetero-junction (BHJ) organic solar cells leads to an ensemble of non-uniform CTE. As a result, the CTE (as well as the PP species) decay non-uniformly by dissociation to free polarons or recombination that deteriorates the cell performance. Empirically, the non-uniform dispersive recombination dynamics in disordered materials have been described [11] by stretched exponential decay in time, or sublinear dependence in the frequency domain [12] , [13] . In this contribution, we address the role of CTE and PP in a number of OPV cells based on BHJ blends, by studying the effect of external magnetic field on their PC response, measured at zero bias. We show that the magneto-PC (MPC) response in such OPV cells has three components; a narrow component, MPC N in fields up to ~0.05 T, an intermediate broad component MPC B up to ~0.7 T and a much broader component, MPC BB that does not saturate even at 8.5 T. We identify the HFI as the main spin-mixing mechanism that explains MPC N ; however, we conclude that the Δ g mechanism [14] in both PP and CTE is the dominant spin-mixing mechanism that explains the two broader MPC components. We further show that the non-Lorentzian MPC( B ) response of the two broad components is caused by the ‘dispersive relaxation’ of the PP and CTE species across the D–A interfaces. MPC measurements The general structure of the OPV cells used in this study is shown in Fig. 1a . 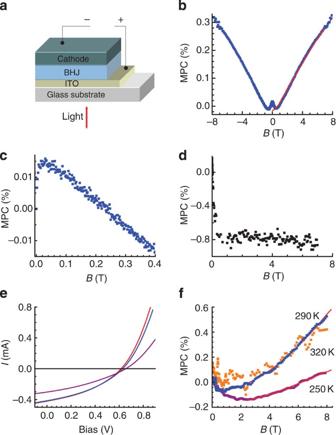Figure 1: High-field MPC of an OPV cell based on D–A blend. (a) An OPV cell structure based on BHJ D–A blend. (b) MPC(B) response of an OPV cell made of rrP3HT/PCBM blend measured at room temperature up to 8 T. The solid line is a fit of the high-field region using the Δgdispersive relaxation model (see text) using the following parameters: ΔB1/2=3.66 T,α=0.74,J/gμB=2.9 mT, Δg=0.002 andτ=0.6 × 10−9s. (c) MPC(B) response showing in more details the field range up to 0.4 T. The solid line is a fit using a HFI+Δgmodel (see text). (d) MC of a diode made of P3HT biased at 3 V using the same set-up as inb. Only the narrow component due to the HFI is obtained. (e,f) I–V characteristics (e) and MPC(B) response (f) of rrP3HT/C61–PCBM (1:1 weight ratio, power conversion efficiency~3%) device, under 470-nm diode laser illumination at various temperatures. The solid red lines through the data points infrepresent fits of the high-field region using the ‘Δgdispersive relaxation’ model (see text). Figure 1b,c shows the MPC( B ) response of a regio-regular P3HT/fullerene blend (rrP3HT/PCBM) OPV cell at room temperature up to 8 T. It reveals three response regions: low-field (| B |<20 mT), where MPC N ( B ) increases with increasing | B | ( Fig. 1c ); intermediate-field (30 mT<| B |<600 mT), where MPC B ( B ) decreases with | B | ( Fig. 1c ); and the high-field region (| B |>0.7 T), where MPC BB ( B ) increases with | B | ( Fig. 1b ). To test the validity of the high-field data, we measured the magneto-conductance response, MC( B ) in a diode made of pristine rrP3HT. The obtained MC( B ) response ( Fig. 1d ) is composed of a narrow negative component (−0.8%), characteristic of spin-mixing due to the HFI that saturates at B 1 ~0.02 T, beyond which the response is flat up to at least 7 T. We thus conclude that the high-field MPC( B ) data shown in Fig. 1b,c,f are not experimental artefacts but rather represent the true response of the OPV cell. The response of the narrow MPC component, MPC N ( B ), has nearly Lorentzian shape with half width at half maximum, HWHM~3 mT, which is characteristic of the HFI constant, a in organic devices [3] , [5] , [6] , [15] . In contrast, MPC B ( B ) and MPC BB ( B ) responses are unlikely to arise from spin-mixing due to the HFI, since a for protons in organics [5] is of the order of a /2 μ B ~3–4 mT ( μ B is the Bohr magneton), much smaller than the field response range of these components. A triplet exciton mechanism [15] , [16] , [17] also cannot account for the broad features, since the typical zero-field-splitting (ZFS) parameter D for triplets in P3HT is of order [18] D /2 μ B ~60–100 mT. We therefore conclude that none of these spin-mixing mechanisms can account for a response that varies strongly beyond B ~600 mT. Figure 1: High-field MPC of an OPV cell based on D–A blend. ( a ) An OPV cell structure based on BHJ D–A blend. ( b ) MPC( B ) response of an OPV cell made of rrP3HT/PCBM blend measured at room temperature up to 8 T. The solid line is a fit of the high-field region using the Δ g dispersive relaxation model (see text) using the following parameters: Δ B 1/2 =3.66 T, α =0.74, J / gμ B =2.9 mT, Δ g =0.002 and τ =0.6 × 10 −9 s. ( c ) MPC( B ) response showing in more details the field range up to 0.4 T. The solid line is a fit using a HFI+Δ g model (see text). ( d ) MC of a diode made of P3HT biased at 3 V using the same set-up as in b . Only the narrow component due to the HFI is obtained. ( e , f ) I–V characteristics ( e ) and MPC( B ) response ( f ) of rrP3HT/C 61 –PCBM (1:1 weight ratio, power conversion efficiency~3%) device, under 470-nm diode laser illumination at various temperatures. The solid red lines through the data points in f represent fits of the high-field region using the ‘Δ g dispersive relaxation’ model (see text). Full size image Figure 1e displays the I–V characteristics of photo-excited rrP3HT/PCBM OPV cell in the temperature range 250–320 K; at lower temperatures the PC is much smaller, mainly due to the decrease in carrier mobility at low temperature. The corresponding MPC( B ) responses are shown in Fig. 1f . It is clearly seen that at 250 K, MPC BB value is smaller than that at 300 K resulting in an increase in the crossover field between the intermediate- (MPC B ) and high-field (MPC BB ) regions (~0.5 versus ~2.5 T). This trend continues at lower temperatures. In addition to the extensive MPC measurements up to ~8 T, we have studied a series OPV cells based on polymer donor–PCBM blend (see Methods for details) on a limited field range. 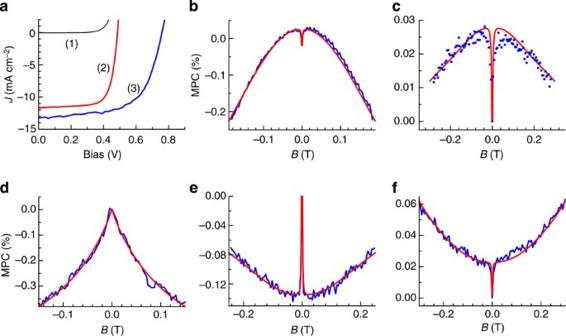Figure 2: MPC of various photovoltaic cells. The MPC(B) response of several bulk hetero-junction OPV cells based on D–A blends of various polymer donors and PCBM, measured at zero bias and room temperature. (a) I–V characteristics measured under the following conditions; (1) dark, (2,3) standard SUN AM1.5 illumination for rrP3HT/C61–PCBM (1.2:1 weight ratio), power conversion efficiency (PCE)=3.2% (2) and PBT7/PC71–BM with 3% dithiol molecules additive, PCE=6.2% (3). (b) MPC(B) response of rrP3HT/PCBM (1.2:1 weight ratio), PCE=3.2%. (c) MPC(B) response for rrP3HT/PCBM (1:1 weight ratio), PCE=1.7%. (d) MPC(B) for PBT7/C71–PCBM with 3% dithiol molecule additives, PCE=6.2%. (e) rraP3HT/C61–PCBM, PCE<1%. (f) MEH-PPV/ C61–PCBM, PCE<1%. The solid red lines through the data points represent simulations to the MPC(B) response using the ‘Δgdispersive relaxation’ model (see text); the fitting parameters are given inSupplementary Table 1. Figure 2a shows representative I–V characteristics of this series, whereas Fig. 2b–f shows their respective MPC( B ) responses, up to ~0.3 T. In this field range, which corresponds to the intermediate field in Fig. 1c , all MPC( B ) responses are characterized by a broad non-saturating component, of which magnitude still varies at the highest field employed. Depending on the polymer donor used, MPC B ( B ) is either decreasing ( Fig. 2b–d ) or increasing ( Fig. 2e,f ) with | B |. The dominant MPC( B ) at low field is the MPC N component due to the HFI having HWHM~3–4 mT ( Fig. 2b,c,e,f ). Figure 2: MPC of various photovoltaic cells. The MPC( B ) response of several bulk hetero-junction OPV cells based on D–A blends of various polymer donors and PCBM, measured at zero bias and room temperature. ( a ) I–V characteristics measured under the following conditions; (1) dark, (2,3) standard SUN AM1.5 illumination for rrP3HT/C 61 –PCBM (1.2:1 weight ratio), power conversion efficiency (PCE)=3.2% (2) and PBT7/PC 71 –BM with 3% dithiol molecules additive, PCE=6.2% (3). ( b ) MPC( B ) response of rrP3HT/PCBM (1.2:1 weight ratio), PCE=3.2%. ( c ) MPC( B ) response for rrP3HT/PCBM (1:1 weight ratio), PCE=1.7%. ( d ) MPC( B ) for PBT7/C 71 –PCBM with 3% dithiol molecule additives, PCE=6.2%. ( e ) rraP3HT/C 61 –PCBM, PCE<1%. ( f ) MEH-PPV/ C 61 –PCBM, PCE<1%. The solid red lines through the data points represent simulations to the MPC( B ) response using the ‘Δ g dispersive relaxation’ model (see text); the fitting parameters are given in Supplementary Table 1 . Full size image To shed light on the origin of the various MPC( B ) components in OPV cells, we have also measured the magneto-photo-induced absorption, MPA, in a film of rrP3HT/PCBM (1.2:1 by weight) blend. 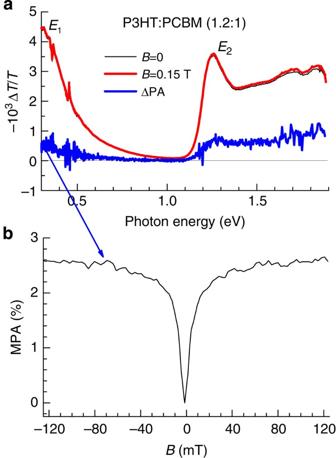Figure 3: MPA of organic D–A blend. (a) PA spectra of a ~100-nm thick film of rrP3HT/PCBM (1.2:1) blend atB=0 (black line) andB=150 mT (red line).E1andE2polaron PA bands are assigned. The difference, ΔPA (enlarged by a factor of 50) is also plotted (blue line). (b) The MPA(B) response obtained atE1=0.35 eV. Figure 3a (black line) displays the measured steady-state photo-induced absorption (PA) spectrum of the film at B =0. The PA is directly related to the steady-state photo-excitation density [19] ; and because of the efficient charge separation in this D–A blend, the PA spectrum primarily shows the long-lived polaron bands that appear here at E 1 ~0.35 eV and E 2 ~1.3 eV, respectively. At B 2 =0.15 T, the PA spectrum ( Fig. 3a , red line) has nearly identical shape as for B =0, but is slightly larger. The difference ΔPA( B 2 )=PA( B 2 )−PA(0) ( Fig. 2a , blue line) is positive, and shows clearly the two polaron bands. The MPA( B ) response measured at the lower-energy polaron band ( E 1 ) that is defined as MPA( B )=ΔPA( B )/PA(0) is shown in Fig. 3b . This response is characterized by a relatively narrow line (HWHM~6 mT) that saturates at B >~50 mT, that is typical to PP magnetic field response in which the HFI is the primary spin-mixing mechanism [5] . We may compare the MPA( B ) response in the blend film with that of MPC( B ) in OPV devices based on the same blend. Since MPA( B ) does not contain a high-field response, we conclude that MPC BB component in MPC( B ) does not originate from long-lived photo-excitations. Therefore, MPC BB must originate from short-lived photo-excited spin-pair, which we identify as CTE species at the D–A interfaces. Figure 3: MPA of organic D–A blend. ( a ) PA spectra of a ~100-nm thick film of rrP3HT/PCBM (1.2:1) blend at B =0 (black line) and B =150 mT (red line). E 1 and E 2 polaron PA bands are assigned. The difference, ΔPA (enlarged by a factor of 50) is also plotted (blue line). ( b ) The MPA( B ) response obtained at E 1 =0.35 eV. Full size image The Δ g mechanism The two broad MPC response components presented in Figs 1 and 2 show that considerable changes in MPC occur in magnetic fields much higher than fields that correspond to the HFI coefficient, a , or triplet ZFS parameters, D and E , or the exchange interaction constant, J . The expected response due to either of these interactions should saturate for |B|>a / gμ B , D / gμ B or J / gμ B , respectively [5] , [20] . For pairs of spins (for example, radical pairs, PP or CTE) that are composed of two spin ½ species with different g -factors, a known spin-mixing mechanism that is more efficient at higher fields is the so-called ‘Δ g mechanism’, where Δ g is the difference in the g -factor of the two spin ½ particles [9] , [21] , [22] . From semi-classical point of view, for B ≠0 the non-identical precession frequencies of the two individual spins in the spin-pair may transform the singlet state to the T 0 triplet state, and vice versa [14] at a rate: Δ ω p =μ B Δ gB / ħ . Thus, the spin-mixing rate, Δ ω p , increases with B ; as a result, if the pair dissociation (or recombination) rate is spin dependent, then consequently the steady-state PC would also vary with B . On the basis of Kaptein theory [23] of spin dynamics in the presence of radical pair diffusion, when taking into account multiple re-encounters of the radicals before their final separation, it was shown [21] that the Δ g –mechanism changes from a Lorentzian profile, in a non-diffusive environment, to a B ½ dependence. It was further shown [22] that, this magnetic field effect (MFE) response saturates at extremely high fields that depend on the parameters of the diffusion kinetics. More recently, the Δ g mechanism was also considered by applying microscopic models of magnetic field effects on charge transport in organic semiconductors [8] , [24] . These latter models were implicitly limited to relatively long decay times, for which the MFE response is mainly determined by the combined effect of the exchange interaction, HFI and Δ g . The active layer in OPV cells is a solid film, and thus the individual spin ½ constituents of the CTE and PP are less likely to diffuse independently, separate and re-encounter many times during the species decay time, τ . Since Kaptein theory is based on multiple re-encounters of charge carriers, we conclude that the Δ g –MFE carrier–diffusion model cannot be applied here for explaining the MPC( B ) response in OPV cells. In addition, the amorphous nature of the organic layer in OPV cells causes a broad distribution of spin-pair species decay times [11] , as has been observed in a variety of electrical, transport [25] and photo-excitation experiments [19] , [26] , [27] . We thus consider an ensemble of static spin-pairs for which the decay mechanism is non-exponential leading to the so-called ‘dispersive relaxation’. We show that in the case of non-dispersive exponential decay, the calculated MPC( B ) response related to the Δ g mechanism is Lorentzian-like with τ -dependent line width. However, dispersive decay (within a non-diffusive static environment) renders the response more concave, in agreement with the experimental results shown in Figs 1 and 2 . Being interested in the MPC( B ) response at fields much larger than the HFI constant, a , we initially ignore the HFI. Consequently, the Hamiltonian for the pair of spin ½ species in a magnetic field may be written as, where J is the exchange interaction coefficient and g i ( g 1 ≠ g 2 ) is the g -factor of spin S i =½ (for simplicity, we assume isotropic exchange interaction response due to and g -tensor). At B =0 the four eigen states may be divided into a singlet (S, at E S =J /2) and a threefold degenerate triplet states (T, at E T =−J /2), see Fig. 4 . For B ≠0 the states are Zeeman separated but only the singlet and T 0 triplet wave functions, ψ S and mix, thereby the spin character of each mixed state becomes B dependent. Specifically, the B -dependent wave functions and energies of the two mixed states at high ( H ) and low ( L ) energies are: , with (Δ ω p =μ B Δ gB / ħ ) as shown in Fig. 4 (see also Supplementary equation (1) ). Thus, starting from an S state at t =0, the S and T 0 populations at any finite field oscillate at the Rabi frequency 2Δ ω p ; this is depicted schematically in Fig. 4 . For a real system with finite lifetime τ , the oscillations are damped, leading to steady-state decay product (for example, free carriers) density of the form: ; this leads to a Lorentzian-type magnetic field response having width Δ B 1/2 ≈ħ /2 μ B Δ gτ . The Lorentzian profile indicates that for a given Δ g , the response saturates at lower fields for species having longer decay times. In particular, the MPC response increases significantly when the decay time, τ , is close to the S–T 0 mixing period (2Δ ω p ) −1 , reaching its full effect at high fields, where the period becomes much shorter than the decay time. In addition, when Δ g is too small (for example, electron–hole pairs in pristine P3HT), then the MFE would be negligibly small, as is the case in Fig. 1d . Formally, to obtain a finite MFE, such as MPC, the bound spin ½ pair must dissociate with decay rate κ that is spin dependent; that is, κ S ≠ κ T [5] , [20] . As B increases from zero, the spin character of each state varies and consequently the overall decay rate also varies with B . It is important to note that κ includes both recombination and dissociation rates, and that the ratio κ S / κ T determines both the sign and magnitude of the specific MFE response; that is, for κ S / κ T >1 the sign is opposite to that of κ S / κ T <1. 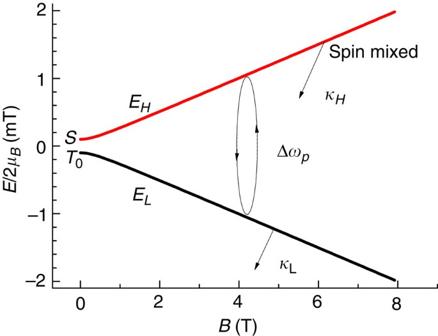Figure 4: Magnetic field-dependent energy levels of spin ½ pair. Evolution with magnetic field of the S/T0states of a pair of spin ½ polarons with differentg-factors (equation (1) withJ/2μB=1 mT, Δg=0.002). AtB=0, the two states are pure S and T0states at energies ±J; forB>0 the states are Zeeman separated and mixed. The effective decay rate of state n=H , L is given by [28] , [29] : Figure 4: Magnetic field-dependent energy levels of spin ½ pair. Evolution with magnetic field of the S/T 0 states of a pair of spin ½ polarons with different g -factors (equation (1) with J /2 μ B =1 mT, Δ g =0.002). At B =0, the two states are pure S and T 0 states at energies ± J ; for B >0 the states are Zeeman separated and mixed. Full size image where is the n th diagonal matrix elements of the projection operator for λ= S or T 0 configuration; note that is B dependent. Using the density matrix formalism, while assuming first-order kinetics, we obtain for the total yield of dissociated carriers (see Supplementary equations (2)–(4) ): where k Dλ is the dissociation rate for λ= S, T, ω n =E n /ħ , the double summation is over all states, ω nm =ω n −ω m , τ nm =1/( γ n + γ m ), and we assume that the photo-excited species are initially in the singlet state [20] , [30] . The most important contribution to the sum in equation (3) comes from the S and T 0 state s for which ω nm ~Δ ω p ≪ | ω T± − ω S |. The MPC( B ) response is given by From equations (3) and (4) we infer that the calculated MPC( B ) response for the Δ g mechanism is Lorentzian-like with HWHM: Δ B 1/2 ≈ħ /2 μ B Δ gτ , where 1/ τ is an average S–T decay rate. In disordered materials such as those used in OPV cells, where decay times are expected to be broadly distributed, we expect ‘dispersive decay kinetics’ having stretched exponential or power law time dependence. For dispersive decay processes the Lorentzian factor in equation (3), namely , may be replaced [13] , [19] by the Cole–Cole function [31] where α ≤1 is the ‘dispersive parameter’ (see Supplementary Discussion , Dispersive relaxation). Small dispersive parameter, α <1 leads to a non-Lorentzian MPC( B ) response that reaches saturation at fields higher than Δ B 1/2 . The implementation of the Cole–Cole function has been proven useful in a variety of experiments such as dielectric spectroscopy [13] and photo-modulation measurements [19] , [26] , [27] , [32] , [33] , where the frequency-dependent products could be well accounted for. As mentioned above, the narrow MPC response component, MPC N ( Figs 1c and 2c ), is due to the HFI within the PP (or CTE) species; this should also be the case for the narrow response shown in Fig. 2b,e,f . For the HFI to be operative, the PP lifetime should be: τ>ħ / a ~2 ns, where a / gμ B ~3 mT is typical strength of the HFI for P3HT. Therefore, PP (or CTE) species having typical lifetime of the order of 0.1 μs (or longer) are the prime candidates responsible for the MPC N response. We note that the g -factors for photo-induced positive and negative polarons in rrP3HT/PCBM blends were measured by light-induced electron spin resonance technique [34] . It was found that g (P + )=2.0017 and g ( P − )=1.9997, leading to Δ g =0.002. Spin-mixing by the Δ g mechanism, which becomes more effective at larger fields, leads to a MFE( B ) response with opposite sign to that caused by the HFI interaction [8] , [9] , that is saturated at high field. We therefore identify the MPC components MPC N and MPC B for | B |<0.4 T, shown in Figs 1c and 2b,c,e , as due to HFI and Δ g mechanism, respectively, of relatively long-lived PP in the BHJ blend. Using the formalism outlined above and in ref. 8 , and assuming dispersive relaxation, the obtained MPC( B ) response shown in Fig. 1c could be simulated with τ =0.1 μs, κ T / κ S =1.05 and α =0.8 (solid line, Fig. 1c ). We note that the narrow component, MPC N , is not always observed ( Fig. 2d ), or it is not opposite to the broad component ( Fig. 2f ). Since for both PP and CTE the HFI should be operative, the observed MPC N is the sum of both contributions. Thus the sign of MPC N is determined by the ratio κ T / κ S in both PP and CTEs, which depends on the specific D–A blend, and therefore may have different sign and magnitude in different blends. We thus conclude that the broad components in MPC( B ) response in Fig. 1 has the same origin as in Fig. 2b–e . In any case the same model (namely HFI and Δ g ) simulates the data in both Figs 1 and 2 very well; the parameters used for the MPC simulations in various OPV devices are given in Supplementary Table 1 . The MPA( B ) response shown in Fig. 3 is dominated by a narrow feature up to B =0.12 T. This is probably due to the preference towards very long-lived PP (PP LL ) in the PA experiment, and consequently also in MPA [8] . These species are probably formed upon P + −P − recombination that occurs in the bulk of the rrP3HT/PCBM blend. Under these conditions, the resulting PP LL are initially in both triplet and singlet spin configurations; in contrast to MPC where the underlying PP are exclusively formed in the singlet configuration. Therefore, since at high fields the T ±1 states of the PP LL do not mix with the S or T 0 states, the contribution of the Δ g mechanism, which is operative only between the S and T 0 states is much weaker. At high magnetic fields and for τ S < τ (where τ S is the spin lattice relaxation time, and τ is the recombination time) the spin PP species may be polarized, or partially polarized at finite temperatures. If the dissociation of the triplet PP (PP T ) is different from that of the singlet PP (PP S ), then the polarized PP system may give rise to a finite contribution to MPC( B ) response of OPV cells. Realizing that the relevant polarizing parameter b=gμ B B / k B T is small ( b ≈0.036 for B =8 T, T =300 K and g =2), we find that the spin polarization contribution to MPC( B ) (namely MPC pol ) is given by the relation (see Supplementary equations (5)–(8) ), where χ = κ T / κ S is the S/T relative contribution to dissociation. From equation (5) it is clear that |MPC pol |< b 2 /4≈0.03% at B =8 T and T =300 K; this is more than an order of magnitude smaller than the observed MPC at room temperature, as shown in Fig. 1b,f . Moreover, b 2 /4 is the maximum value for MPC pol and is obtained only for the extreme case where 1/ χ =0 and τ s / τ =0. In reality, however, χ is of order 1 (typically, |1− χ |<0.1, see above and refs 5 , 15 ), and the decay time τ is not necessarily longer than τ s , especially for CTE where τ < τ s . Thus, the calculated MPC pol at room temperature may be two or more orders of magnitude smaller than the measured MPC. In addition, equation (5) predicts an increase in MPC magnitude as the temperature decreases, because b increases at low T . In contrast, Fig. 1f shows that the obtained MPC BB behaves in an opposite way: namely, its magnitude decreases with decreasing temperature from 320 to 250 K (this trend continues at lower temperatures). We therefore conclude that the observed MPC BB at T ≥250 K is not caused by magnetic field-induced spin polarization. This effect, however, might be important at cryogenic temperatures [10] . We therefore conclude that the Δ g mechanism is the only spin-mixing mechanism that may explain the high-field and room temperature component, MPC BB (| B |>0.6 T), where MPC BB ( B ) increases with | B | ( Fig. 1b,f ). To explain the large MPC BB ( B ) response in this region the spin ½ pair lifetime should be short. The fact that MPC BB ( B ) response increases monotonically with B and does not saturate up to ~8.5 T implies an effective decay time of <~1 ns. This strongly indicates that CTE species are responsible for the MPC BB component. Indeed, recent studies revealed that CTE at the D–A interface dissociate into free polarons in rrP3HT/PCBM blend on a sub-nanosecond timescale [35] . Also, the apparent non-Lorentzian shape of MPC BB ( B ) points towards ‘dispersive relaxation’, as discussed above. The solid line in Fig. 1b is a fit to the data using the Δ g mechanism (equations (1)–(4)) with dispersive relaxation; the best-fitting parameters for this fit are: α =0.7, κ T / κ S =0.95, τ =0.6 ns. However, these latter parameters are device dependent; for the device shown in Fig. 1f , the best-fitting parameters that we obtained are: α =0.8–0.9, κ T / κ S ~0.95, τ =0.2–0.4 ns. Note that, whereas MPC B ( B ) due to PP decreases with increasing field, MPC BB ( B ) due to CTE increases with increasing field. The MPC value and polarity are determined by a delicate balance between the singlet and triplet spin sublevel dissociation yields. If both κ S =κ T and the S/T dissociation rates k DS =k DT , then MPC=0. Slight variations in the recombination rates and in the ratios κ T / κ S and/or k DT / k DS may change significantly the MPC value and polarity. Such variations may occur, for example, due to morphology, carrier mobility, contamination (oxygen, humidity), photo-excitation intensity and so on. We believe that this environmental sensitivity explains the different MPC B and MPC BB polarities seen in Figs 1 and 2 . Devices and materials A solvent–cast layer of an organic donor and 1-[3-(methoxycarbonyl)propyl]-1-1-phenyl)[6,6]C 60 (PCBM) acceptor blend was sandwiched between the cathode (for example, Ca covered by Al film) and the transparent anode (film of indium tin oxide, ITO) through which the active layer was photo-excited; the general structure of the OPV cells used is shown in Fig. 1a . We used several different donor polymers obtained from various sources, which include: regio-regular poly(3-hexylthiophene) (rrP3HT), regio-random P3HT (rraP3HT), thieno[3,4- b ] thiophene/benzodithiophene (PTB7) with and without dithiol molecule additives [36] , and poly[2-methoxy-5-(2-ethylhexyloxy)-1,4-phenylenevinylene] (MEH-PPV). These blends are known to form BHJ of nano-sized domains that facilitate charge photogeneration, transport and collection in the active layer of the cell. The power conversion efficiency of the OPV cells based on the D–A blends varied between 0.5 and 6%, depending on the polymer donor. PC and MPC measurements The I–V and MPC measurements were performed at various temperatures under constant bias, V b . A variety of I–V characteristics in the dark and under illumination are shown in Figs 1e and 2a for representative cells. For measurements in a magnetic field we used electrical wires made of metallic alloys to keep the parasitic magneto-resistance below 0.001%. For the MPC measurements, the OPV devices were transferred to a cryostat that was placed in a magnetic field B . For the temperature-dependent measurements, the temperature was controlled to better than ±0.2 K to prevent unwanted changes in the short circuit current. The magnetic field was provided by an electromagnet with B up to 0.45 T, or a superconducting magnet with B up to ~8.5 T. The OPV devices were illuminated with a tungsten lamp or a UV–visible light emitting diode, and the PC was measured at zero bias ( V b =0) while sweeping the external magnetic field in one direction and back for several cycles to improve the signal-to-noise ratio ratio. MPC is defined as MPC( B )=[PC( B )/PC(0)−1], where PC is the short circuit current under illumination. How to cite this article: Devir-Wolfman, A. H. et al. Short-lived charge-transfer excitons in organic photovoltaic cells studied by high-field magneto-photocurrent. Nat. Commun. 5:4529 doi: 10.1038/ncomms5529 (2014).